Ultrafast direct modulation of a single-mode photonic crystal nanocavity light-emitting diode Low-power and electrically controlled optical sources are vital for next generation optical interconnect systems to meet strict energy demands. Current optical transmitters consisting of high-threshold lasers plus external modulators consume far too much power to be competitive with future electrical interconnects. Here we demonstrate a directly modulated photonic crystal nanocavity light-emitting diode (LED) with 10 GHz modulation speed and less than 1 fJ per bit energy of operation, which is orders of magnitude lower than previous solutions. The device is electrically controlled and operates at room temperature, while the high modulation speed results from the fast relaxation of the quantum dots used as the active material. By virtue of possessing a small mode volume, our LED is intrinsically single mode and, therefore, useful for communicating information over a single narrowband channel. The demonstrated device is a major step forward in providing practical low-power and integrable sources for on-chip photonics. Optical interconnects have attracted much research attention in recent years owing to potential performance and power-consumption improvements over traditional electrical connectivity. A complete optical interconnect link consists of a modulated optical source, passive components to route light, a photodiode for detection, and driving circuitry. To be a viable solution for next-generation systems, the complete energy budget for an optical link should be about 10 fJ per bit, while the operating speed should be at least 10 GHz (ref. 1 ). Unfortunately, previously demonstrated laser sources have μW to mW thresholds and the best external modulators consume 100 s of fJ to pJ per bit level energies [2] , [3] , [4] . Alternative to the standard approach of using a continuous wave laser and external modulator, direct modulation of a fast optical source can drastically reduce the energy consumption for the transmitter. A recent demonstration of all optical switching of a photonic crystal (PC) cavity laser showed fast 20 Gb s −1 switching at low power, corresponding to an energy of only 8.76 fJ per bit (ref. 5 ). This technique relied, however, on optical pumping, and is difficult for on-chip integration. Recently, we demonstrated an electrically driven photonic crystal quantum dot (QD) nanocavity laser with world record low threshold of 208 nW based on a lateral p-i-n junction defined by ion implantation in gallium arsenide [6] . This electrical pumping scheme allows for efficient current injection into the intrinsic cavity region [7] , [8] . Controlling photonic crystal cavities electrically leverages their advantages such as low-power and single-mode emission while maintaining practical integration. The demonstrated nanolasers operate at temperatures up to 150 K before transitioning to single-mode light-emitting diode (LED) operation at room temperature because of reduced quantum dot gain. Although power output is smaller in the LED regime, it is still in the range usable for optical interconnects where sensitive photodetectors exist [9] ; moreover, we are able to exploit the fast switching properties of single-mode output from a nanocavity. In this work, we show that we are able to electrically switch such a single-mode photonic crystal nanocavity LED at 10 GHz speed and at room temperature with electrical injection power at the μW level. As a photonic crystal cavity has only a few unique modes in spectrally distant locations, our diode is effectively a single-mode light source and can be used as a fast, low-power transmitter for optical interconnects. 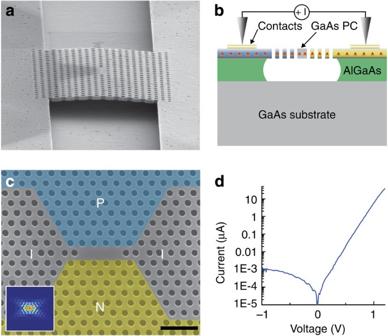Figure 1: Schematic of electrically pumped photonic crystal cavity devices. (a) Tilted scanning electron microscope image of a device. The doping profile is partially visible in the picture. (b) Vertical cross-section layout of device structure. Quantum dots are represented as triangles. (c) Top-down scanning electron microsope view of a photonic crystal membrane highlighting the approximate boundaries of the doping areas. The figure is oriented 90 degrees clockwise compared with (a). The inset is the fundamental cavity mode electric field amplitude as calculated from finite-difference time domain. The scale bar is 1 μm. (d) Diode current-voltage plot measured for a typical LED device. Device design and LED operation Figure 1a–c shows a schematic of a fully fabricated photonic crystal cavity LED. A series of ion implant steps through a silicon nitride mask defined the lateral p-i-n junction in a 220-nm thick GaAs membrane with embedded high-density quantum dots, as in our previous work [6] . After an activation anneal for the dopants, photonic crystals were patterned and transferred to the membrane through a dry etch step. Metal contacts were then deposited and the sacrificial AlGaAs layer beneath the GaAs membrane was wet-etched to release the photonic crystal structures. We chose a modified L3 defect cavity design [10] with a fundamental mode wavelength within the inhomogeneous distribution of the QD ensemble, centred near 1,230 nm at room temperature. The fundamental mode for this cavity design (inset in Fig. 1c ) has a theoretical quality factor in excess of 10 5 , as calculated from finite-difference time domain simulations. Figure 1: Schematic of electrically pumped photonic crystal cavity devices. ( a ) Tilted scanning electron microscope image of a device. The doping profile is partially visible in the picture. ( b ) Vertical cross-section layout of device structure. Quantum dots are represented as triangles. ( c ) Top-down scanning electron microsope view of a photonic crystal membrane highlighting the approximate boundaries of the doping areas. The figure is oriented 90 degrees clockwise compared with ( a ). The inset is the fundamental cavity mode electric field amplitude as calculated from finite-difference time domain. The scale bar is 1 μm. ( d ) Diode current-voltage plot measured for a typical LED device. Full size image The measured current–voltage characteristics for a device are shown in Figure 1d . Our LED has robust electrical properties with over three orders of magnitude on/off ratio and minimal leakage current. In contrast to the laser diode in our earlier work [6] , we have eliminated the substrate leakage path by oxidizing the sacrificial layer for a longer time (Methods) and now all of the current travels through the PC membrane. Only 3–4% of the current is estimated to leak through the wide intrinsic region mirrors of the device, with the remaining 96–97% flowing through the cavity. The measured series resistance of 1.3 kΩ is mostly due to the sheet resistance of the thin membrane, modified by the air hole fill factor that decreases the effective current cross-section [11] . 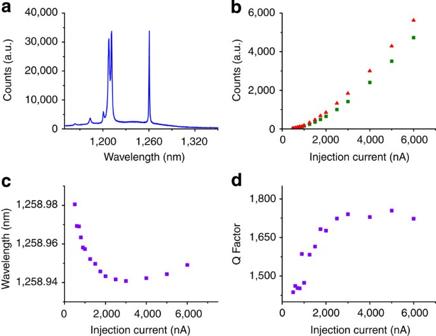Figure 2: Optical properties of LEDs under DC bias. (a) Spectrum of the cavity for a forward bias current of 10 μA. (b) Current-light output plot for both the fundamental cavity mode (red triangles) at 1,259 nm and uncoupled background spontaneous emission (green squares). (c) Peak wavelength of the cavity mode versus injection current. (d) Fundamental mode quality factor versus injection current. A spectrum of the emission for the LED from Figure 1 is shown in Figure 2a at a forward bias current of 10 μA and at room temperature. Bright and clearly defined cavity modes peak well above the background QD emission with the fundamental mode centred at 1,259 nm. As the pump current increases, the intensity of the fundamental mode emission increases superlinearly ( Fig. 2b ); however, room-temperature lasing can be ruled out, because the spontaneous emission intensity uncoupled to the cavity also follows the same trend, in contrast to our prior reported laser at low temperature [6] . Possible explanations for the superlinear emission behaviour are an increase in QD emission efficiency with increasing carrier density [12] as well as multiexcitonic effects from higher order QD states [13] ; considering that the same superlinear emission behaviour is observed at all wavelengths, we believe that this is a result of the former effect [12] . The peak wavelength of the cavity mode shown in Figure 2c is first seen to blueshift because of free carrier dispersion before redshifting at high biases. The magnitude of the blueshift ~40 pm corresponds to an injected carrier level of 10 16 cm −3 , in good agreement with simulations, and the slight redshift for higher biases indicates a sample self-heating of at most a few degree Celsius. Figure 2d shows the cavity quality (Q) factor versus injection current and demonstrates that, even at room temperature, a small amount of gain from the quantum dots is observed. The reduction in QD gain at room temperature compared with cryogenic temperatures is ascribed to modified properties of our quantum dots after rapid thermal annealing, described in the next section. Figure 2: Optical properties of LEDs under DC bias. ( a ) Spectrum of the cavity for a forward bias current of 10 μA. ( b ) Current-light output plot for both the fundamental cavity mode (red triangles) at 1,259 nm and uncoupled background spontaneous emission (green squares). ( c ) Peak wavelength of the cavity mode versus injection current. ( d ) Fundamental mode quality factor versus injection current. Full size image Lifetime measurements To better understand the system, we employ a three-level rate equation model and experimentally measure various lifetime processes [14] . The coupled rate equations are as follows: The free carrier and quantum dot carrier densities are given by N B and N QD , respectively. V is the active pumped volume and q is the electron charge. Free carriers are injected into the upper level through a pump current, I , and then decay either radiatively (rate 1/ τ SP,B ), nonradiatively (rate 1/ τ NR ), or into the quantum dots (rate 1/τ C ). The captured carriers in the quantum dots can then either recombine through Purcell-enhanced spontaneous emission at rate F C / τ SP,QD (where F C is the Purcell factor and 1/ τ SP,QD is the ordinary spontaneous emission rate) or be reemitted back into the free carrier upper level at rate 1/ τ E . We neglect any stimulated emission term in the rate equations as our diode is non-lasing. At cryogenic temperatures, the InAs quantum dots have a long (>1 ns) bulk lifetime due to the trapping of carriers inside the QD confining potential (negligible N QD / τ E rate). Near room temperature, however, the thermal energy of trapped carriers allows for a non-zero reemission rate (that is, shorter τ E ) and a lower overall QD lifetime of around 100–300 ps due to bulk nonradiative recombination ( Supplementary Fig. S1 ). In our devices, the quantum dots undergo a rapid thermal annealing step at 850 °C to activate the nearby implanted dopants. This high-temperature step causes the QD ensemble emission to blueshift by 80 nm and spectrally broaden ( Fig. 3a ). Probably, the QD core intermixes with the wetting layer and there is a narrowing of the overall QD sizes, as seen previously [15] . These effects would suggest a shallower confining potential and, hence, a more rapid reemission of carriers from the quantum dots. If, in addition, there is fast nonradiative recombination present (that is, short τ NR resulting from etched GaAs surfaces), the overall lifetime and emission strength of the quantum dots should be reduced because of thermal escape and quenching. 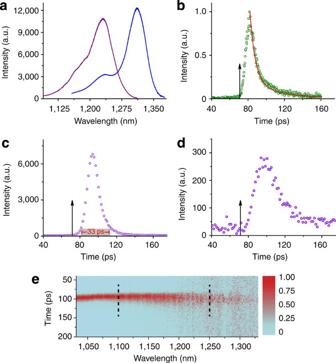Figure 3: Optically pumped time-resolved measurements of annealed sample. (a) Bulk QD photoluminescence spectrum under continuous wave pumping for post- (left) and pre- (right) annealed samples. (b) GaAs band edge emission at 870 nm from the photonic crystal region. The vertical arrow represents the optical pump pulse and the solid line is a fit to the experimental data giving a 6-ps dominant exponential decay term. (c) Quantum dot lifetime at 1,100 nm under equivalent excitation as in (b). The grey box indicates the QD emission intensity that is greater than 10%, giving an effective pulse duration of 33 ps. (d) QD lifetime at 1,250 nm, exhibiting an 18 ps fall time. (e) Spectrum of room temperature lifetime data for the broad range of QD emission wavelengths. To clarify the data due to the poor sensitivity of the detector for longer wavelengths, intensities have been normalized in 3 nm bins. Vertical dashed lines indicate slices from which (c) and (d) have been taken. Figure 3: Optically pumped time-resolved measurements of annealed sample. ( a ) Bulk QD photoluminescence spectrum under continuous wave pumping for post- (left) and pre- (right) annealed samples. ( b ) GaAs band edge emission at 870 nm from the photonic crystal region. The vertical arrow represents the optical pump pulse and the solid line is a fit to the experimental data giving a 6-ps dominant exponential decay term. ( c ) Quantum dot lifetime at 1,100 nm under equivalent excitation as in ( b ). The grey box indicates the QD emission intensity that is greater than 10%, giving an effective pulse duration of 33 ps. ( d ) QD lifetime at 1,250 nm, exhibiting an 18 ps fall time. ( e ) Spectrum of room temperature lifetime data for the broad range of QD emission wavelengths. To clarify the data due to the poor sensitivity of the detector for longer wavelengths, intensities have been normalized in 3 nm bins. Vertical dashed lines indicate slices from which ( c ) and ( d ) have been taken. Full size image To confirm this hypothesis, we perform time-resolved photoluminescence measurements of our post-annealed sample using a mode-locked Ti:Sapphire laser for excitation and a streak camera with an extended range detector unit. The free carrier nonradiative recombination rate can be measured by examining the behaviour of the 870-nm GaAs band edge emission in a photonic crystal region. Figure 3b shows that the nonradiative lifetime, τ NR , in a PC region is very short at 6 ps because of the presence of many etched-hole surfaces [16] . Meanwhile, the measured QD lifetime is only 10 ps at 1,100 nm ( Fig. 3c ), far shorter than the 100–300 ps result for pre-annealed samples ( Supplementary Fig. S1 ) and thus verifying the rapid carrier escape prediction. This result means that luminescence from quantum dots can effectively be turned off in ~10 ps, with ~4 ps attributed to the carrier reemission time ( τ E ) and 6 ps to the nonradiative surface recombination. For longer wavelength QDs, the turn-off time slowly increases monotonically with wavelength indicating deeper carrier confinement ( Fig. 3d,e ). The QD carrier capture time ( τ C ) can be estimated from the leading edge of the QD emission and is 10 ps. Therefore, the QD turn on time is approximately the sum of this term plus the rise time for free carriers (also 6 ps) for a total time of 16 ps. As seen in Figure 3c, the time duration for which the QD emission pulse is greater than 10% is only 33 ps. Consequently, our LED is capable of switching speeds of up to 30 GHz. Direct electrical modulation We next perform time-resolved direct electrical modulation studies to determine the electrical response of our devices. As our detector has two orders of magnitude better sensitivity at 1,100 nm compared with the QD peak gain at 1,230 nm, we examine a different cavity than the one shown in Figure 2 . Although this wavelength corresponds to excited states of the quantum dots, the switching lifetimes are still governed by the same rapid carrier escape effects. The only difference between QD transitions at 1,100 nm and 1,230 nm is a shallower carrier confinement at shorter wavelength and therefore slightly faster turn-off time. 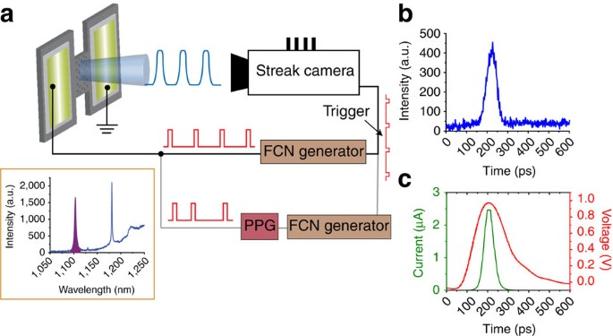Figure 4: Experimental set-up and results for electrical modulation of the nano-LED. (a) Schematic for the direct modulation experiments. For a single-pulse time-resolved measurement, only the function (FCN) generator is used (black path) whereas for multiple pulses a pulsed pattern generator (PPG) is also used (grey path). Inset shows the emission spectrum for the cavity used in direct modulation experiments. The filled in peak is the isolated mode at 1,100 nm. (b) The output optical pulse measured when the LED is driven by the pulse shown in (c). (c) Driving voltage and current pulses for the measurement in (b). The peak power is only 2.5 μW. As seen in the inset of Figure 4a , this cavity has a bright higher order mode at 1,100 nm despite the low background QD emission in that spectral region. The Q factor for this mode is lower than for the fundamental mode and is measured to be 250. Similar to the cavity mode in Figure 2 , the mode at 1,100 nm also exhibits a superlinear pump power dependence and minor linewidth narrowing. The experimental set-up consists of the same streak camera detector as before; however, instead of an 80-MHz optical pump, we use an 80-MHz electrical pulse generator to drive the LED directly ( Fig. 4a ). For single-shot measurements, we use only a regular function generator while, for pulse train measurements, a pulse pattern generator is used in conjunction with the first function generator. To ensure proper signal referencing of the LED and detector, the two electrical sources are clocked together (see Methods ). Figure 4: Experimental set-up and results for electrical modulation of the nano-LED. ( a ) Schematic for the direct modulation experiments. For a single-pulse time-resolved measurement, only the function (FCN) generator is used (black path) whereas for multiple pulses a pulsed pattern generator (PPG) is also used (grey path). Inset shows the emission spectrum for the cavity used in direct modulation experiments. The filled in peak is the isolated mode at 1,100 nm. ( b ) The output optical pulse measured when the LED is driven by the pulse shown in ( c ). ( c ) Driving voltage and current pulses for the measurement in ( b ). The peak power is only 2.5 μW. Full size image In Figure 4b, we see the ultrafast response of our LED when a short electrical pulse is applied. Although the voltage pulse has a full-width at half-maximum of over 200 ps, the injected current is highly nonlinear with voltage and hence the pump current pulse is quite narrow at 60 ps full-width at half-maximum ( Fig. 4c ). The resultant single-mode diode response tracks the current pulse nicely after an initial turn on delay. This result demonstrates that our single-mode LED device is indeed capable of ultra-fast electrical switching at many GHz speed. The entire pulse duration (the time above 10% of the peak height) is less than 100 ps and, therefore, the LED switching speed for a non-return-to-zero signal is ~10 GHz. Compared with previously shown directly modulated photonic crystal single-mode LEDs at cryogenic temperatures [17] , this speed is over an order of magnitude faster with three orders of magnitude lower power consumption (here only 2.5 μW). It is interesting to note that the photonic crystal RC time constant does not impact the diode response at these speeds because of the incredibly small capacitance of the p-i-n junction ( Supplementary Methods ). For this particular cavity at room temperature, we do not quantitatively observe Purcell enhancement due to the dominant carrier escape rate over the spontaneous emission rate. Next, we directly modulate our diode with a pulse train to observe dynamic behaviour with a multiple bit sequence. To do this, a programmed bit stream from a pulsed pattern generator is applied to the LED while the other function generator sends a triggering signal to the streak camera (see Methods ). 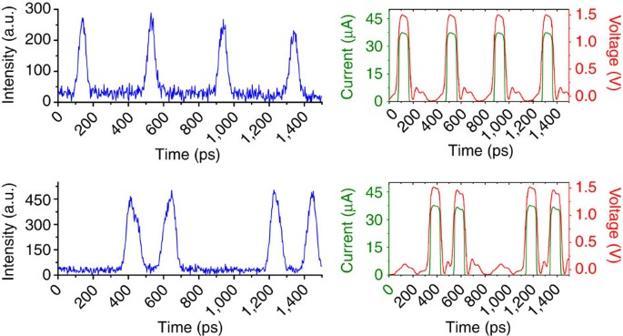Figure 5: Direct electrical modulation of photonic crystal LED. Diode response for two different bit sequences in top and bottom panels. The applied electrical voltage and current are shown on the right and the LED optical output is on the left. Figure 5 shows the light output for two different bit sequences, along with corresponding pump signal data. The diode replicates the bit sequences well and behaves very much like the single-shot measurement above. On-pulses are still about 100 ps wide and the bit stream has clearly resolvable off-pulse sections. Fast electrical data is thereby effectively mapped onto the single-mode carrier of the nanocavity LED, which can be used as the light source for an optical interconnect link. Figure 5: Direct electrical modulation of photonic crystal LED. Diode response for two different bit sequences in top and bottom panels. The applied electrical voltage and current are shown on the right and the LED optical output is on the left. Full size image The results presented here show, for the first time, GHz speed direct electrical modulation of a single-mode LED at ultra-low energies. In fact, the measured power consumption for the 10 GHz pulse in Figure 4 is only 2.5 μW, indicating an average energy per bit of only 0.25 fJ. This exceptionally low value indicates significant improvement over the standard approach of using slow, high-threshold lasers and external modulator components. For example, typical 'low' power ring-based modulators require an average energy per bit of ~500 fJ whereas MZI modulators have pJ switching energies [4] , [18] . Information can just as easily be communicated over a directly modulated low-power source, skipping the external modulator altogether. Furthermore, chirp is a non-issue for directly modulated LED, because optical interconnect distances are so short that dispersion of pulse data can be neglected. This new paradigm of replacing traditional power-hungry lasers and modulators with ultrafast nanocavity light sources could allow optical interconnects to meet the energy targets needed for wide-scale adoption. Our PC LED has one of the fastest switching speeds ever demonstrated for an LED device, either low-power and single-mode or high-power and multimode. Other researchers have previously demonstrated a record LED −3 dB cutoff speed at 7 GHz using a bipolar junction to sweep away carriers that do not recombine fast enough [19] . Although we do not explicitly measure a −3-dB point, a single-pole analysis of the 10 ps turn-off time found above for QDs at 1,100 nm suggests a very large −3 dB bandwidth of 16 GHz. The single-mode operation of our diode at low power, however, is far more attractive for on-chip communications than the previously demonstrated high-speed LED [19] . We find the output power for our device to be 10 s to 100 s of pW at μW bias levels, indicating an efficiency of ~10 −5 ( Supplementary Methods ). This result is not surprising given the fact that the majority of carrier recombination is nonradiative and not through QD emission. Nonetheless, such low-power signals can be detected using advanced photodetector technologies. For example, various nanoscale avalanche photodiodes have been demonstrated in different material systems that can effectively detect low-level (even sub-pW) signals [9] , [20] , [21] . Another promising strategy for improving the responsivity of near-infrared photodetectors is via plasmonic concentration of light with resonant antennas or metallic structures [22] , [23] . It has been proposed that single-mode LEDs can have very high modulation bandwidths under situations where the spontaneous emission rate is increased through Purcell enhancement alone [24] . In this scenario, quantum efficiencies could be made higher because the predominant recombination process is radiative. Meanwhile, the modulation bandwidth is boosted by the ability to speed up LED spontaneous emission through cavity enhancement. We examine the tested device from Figure 4 at 10 K temperature and perform time-resolved studies on the quantum dot emission lifetimes. As shown in the Supplementary Discussion , we find that the cavity emission lifetime at 1,100 nm is decreased threefold compared with uncoupled QD emission, corresponding to a Purcell factor of 5.5 ( Supplementary Fig. S2 ). Therefore, our device could utilize Purcell enhancement for fast switching at cryogenic temperatures where carrier escape and nonradiative recombination effects are minimized. In contrast, at room temperature, thermal excitation of carriers depopulates the quantum dots much quicker than does Purcell-enhanced spontaneous emission, and modulation time is thus limited by nonradiative effects, as a result of material issues. Our experimental studies shown in Supplementary Figure S3 reflect this conclusion, because QD emission off-resonant with the cavity mode decays just as quickly as does on-resonant emission. This limitation is a fundamental material constraint for these types of quantum dots inside GaAs and is not due to our fabrication process or device design, as explained in the Supplementary Discussion . We believe that fast switching realized by Purcell enhancement alone could be accomplished by shutting down nonradiative recombination completely, which would require using quantum dots with deeper confining potentials, combined with sophisticated surface passivation techniques, or use of a different material system (such as InP-based) with lower surface recombination rates [25] . We emphasize that despite the device speed not being Purcell-factor limited, the presence of the nanocavity in our LED has several great benefits, including the improvement of the device efficiency (increased light emission into the cavity mode and channelling of photons in the desired, collection direction), the reduction in the modulation energy per bit, and single-mode operation, which is critical for optical interconnect applications [1] . In summary, we have demonstrated an ultrafast single-mode nanocavity LED operating at room temperature with 10-GHz large signal direct modulation speed. A lateral p-i-n photonic crystal diode provides extremely low modulation energies of fJ per bit, and can be readily applied to other III–V materials with different gain media and surface properties, leading to a large range of possible device characteristics. The low energy per bit of these optical sources makes them promising for future energy-efficient optical interconnect applications. Fabrication Devices were fabricated using an identical process, as described before [6] , with the exception that the thermal oxidation was increased to 15 min to complete the sacrificial layer oxidation. Cavities were fabricated to have a range of lattice constants, a =300–340 nm, and hole radii, r / a =0.2–0.25. The devices tested had a =330 nm and r =65 nm. Optical testing Samples were mounted on a stage at room temperature and contacted directly by low-speed electrical probes. A source meter with sub-nano-amp accuracy was used to drive devices. Emission was collected by a 0.5 NA objective lens and directed toward a spectrometer with a liquid-nitrogen-cooled InGaAs charge-coupled device detector. Cryogenic testing was performed by mounting samples inside a helium-flow cryostat. High-speed measurements Time-resolved optical testing was performed using an 80-MHz Ti:Sapphire laser generating 3-ps width pulses. The samples were mounted and the collected photoluminescence was detected by a Hamamatsu C5680 streak camera with 2 ps resolution. For time-resolved electrical measurements, the devices were contacted by high-speed probes having a 40-GHz cutoff frequency. An Agilent 8133A function generator was used to drive both the LED device and streak camera at 80 MHz for single-pulse measurements. To perform pulse train experiments, an Anritsu MP1800A pulse pattern generator was used to program a bit pattern that was sent to the LED device. This pattern length had a repetition rate faster than the 80 MHz required by the streak camera for locking. It was sent to the Agilent function generator, where it was divided by an integer number such that the repetition rate of the new signal was close to 80 MHz. This new signal provided the proper trigger for the streak camera and was clocked correctly with the original drive signal. How to cite this article: Shambat, G. et al . Ultrafast direct modulation of a single-mode photonic crystal nanocavity light-emitting diode. Nat. Commun. 2:539 doi: 10.1038/ncomms1543 (2011).